The locust genome provides insight into swarm formation and long-distance flight Locusts are one of the world’s most destructive agricultural pests and represent a useful model system in entomology. Here we present a draft 6.5 Gb genome sequence of Locusta migratoria , which is the largest animal genome sequenced so far. Our findings indicate that the large genome size of L. migratoria is likely to be because of transposable element proliferation combined with slow rates of loss for these elements. Methylome and transcriptome analyses reveal complex regulatory mechanisms involved in microtubule dynamic-mediated synapse plasticity during phase change. We find significant expansion of gene families associated with energy consumption and detoxification, consistent with long-distance flight capacity and phytophagy. We report hundreds of potential insecticide target genes, including cys-loop ligand-gated ion channels, G-protein-coupled receptors and lethal genes. The L. migratoria genome sequence offers new insights into the biology and sustainable management of this pest species, and will promote its wide use as a model system. Since the dawn of agrarian civilization, locust plagues have been viewed as one of the most devastating natural disasters, linked with famine, strife and dissolution of societal order as documented in the Bible, the Qur’an and Chinese historical records [1] , [2] . Unfortunately, locust plagues continue to cause destruction even today. For example, in 1988, locust swarms covered an enormous area of some 29 million square kilometres, extending over or into parts of up to 60 countries, resulting in billions of dollars in economic losses [3] . The primary current method for combating locust outbreaks is through intensive spraying of chemical pesticides; however, their overall usefulness has been widely debated because of their highly negative impact on human and environmental health, and on biological diversity [2] . Locusts are grasshopper species with swarming and long-distance migratory behaviours [1] . Locust swarms form suddenly and unpredictably through the congregation of billions of insects, which can fly hundreds of kilometres each day, and even cross oceans [4] . They are polyphagous and a single individual consumes its own body weight in food in 1 day; this is, proportionately, 60–100 times a human’s daily consumption [1] . Locusts are characterized by a density-dependent phase polyphenism, which involves a variety of biological and phenotypic traits, including changes in body colour, morphology, behaviour, physiology, immune responsiveness and others [5] , [6] , [7] , [8] , [9] . An increase in population density triggers the transformation from a well-hidden solitarious phase to an overtly noticeable gregarious phase, which results in an extensive aggregation of individuals [1] . This phase change occurs quickly and reversibly, and its speed varies among species [10] . The entire transformation process of phase change pivots around a behavioural change, which has been proposed to be regulated by the peripheral and central nervous system (CNS) [11] , [12] , [13] . The migratory locust, Locusta migratoria , is the most widespread locust species and has long served as a model organism for insect morphology, behaviour and physiological research [14] , [15] , [16] . Here we provide a draft genome sequence of L. migratoria , the largest animal genome sequenced so far. We assess changes of gene families related to long-distance migration, feeding and other biological processes unique to the locust and identify genes that might serve as potential pesticide targets. Combining a set of transcriptome and methylome data from gregarious and solitarious locusts, we reveal potential neuronal regulatory mechanisms underlying phase change in the locust. Genome assembly We sequenced the genome of a single, eight-generation inbred female individual of L. migratoria , worldwide distributed agricultural pests ( Supplementary Fig. S1 ), using the Illumina HiSeq 2000 sequencing platform. After quality control and filtering, 721 Gb of data were generated, covering 114 × of the 6.3 Gb L. migratoria genome size as estimated by k -mer analysis and flow cytometry ( Supplementary Tables S1 and S2 , and Supplementary Figs S2 and S3 ). We used SOAPdenovo [17] to perform de novo assembly, achieving a final assembly of 6.5 Gb with a length-weighted median (N50) contig size of 9.3 kb and scaffold N50 of 320.3 kb ( Supplementary Table S3 ). A genetic map containing 11 major linkage groups was further developed based on 8,708 markers using restriction-site-associated DNA sequencing data ( Fig. 1a ). 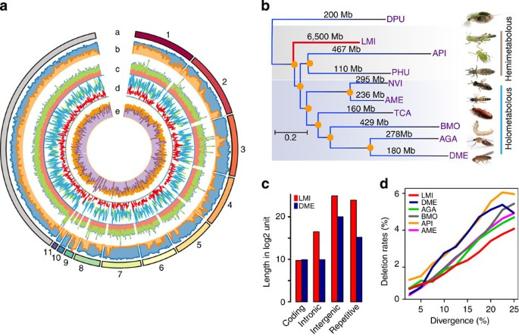Figure 1: Locust genomic characterization and comparative analysis of insect genomes. (a) A schematic representation of genomic characteristics of the locust pseudo-chromosomes (in an Mb scale). Track a: 11 linkage groups of the locust genome, grey denotes unmapped scaffolds. Track b: coverage of sequencing depth (blue) and distribution of allelic heterozygous single-nucleotide polymorphisms (SNPs) between the two haploids (orange). Track c: density distribution of three dominant subclasses of repetitive element (DNA transposons, red; LINEs, green; long terminal repeats (LTRs), blue). Track d: divergence rates of three dominant subclasses of repetitive element (DNA transposons, red; LINEs, green; LTRs, blue). Track e: ratio of observed to expected frequency of CpG dinucleotides in the coding region of gene sets (orange) and in the whole genomic region (violet). (b) Phylogenetic relationships inferred based on the concatenated data set from universal single-copy genes. The number in the branches indicates the genome sizes. (c) Size expansion of genomic components of a homologous and syntenic locus between the locust and fly genome inferred from theOsirisgenes, a conserved gene family across insects. (d) Deletion rates across five insect genomes that contain a substantial fraction of LTR retrotransposon copies. Because of their relaxed selection pressures and reputed neutral decay rates, LTR retrotransposon copies were used to estimate deletion rates. RepeatMasker searches were performed to determine the deletion rates of genomic retrotransposon copies using intact LTR retrotransposons as a query. The genomic visualization was created using the programme Circos. AGA,A. gambiae; AME,A. mellifera; API,A. pisum; BMO,B. mori; DME,D. melanogaster; DPU,D. pulex; LMI,L. migratoria; NVI,Nasonia vitripennis; PHU,P. humanus; TCA,Tribolium castaneum; . Figure 1: Locust genomic characterization and comparative analysis of insect genomes. ( a ) A schematic representation of genomic characteristics of the locust pseudo-chromosomes (in an Mb scale). Track a: 11 linkage groups of the locust genome, grey denotes unmapped scaffolds. Track b: coverage of sequencing depth (blue) and distribution of allelic heterozygous single-nucleotide polymorphisms (SNPs) between the two haploids (orange). Track c: density distribution of three dominant subclasses of repetitive element (DNA transposons, red; LINEs, green; long terminal repeats (LTRs), blue). Track d: divergence rates of three dominant subclasses of repetitive element (DNA transposons, red; LINEs, green; LTRs, blue). Track e: ratio of observed to expected frequency of CpG dinucleotides in the coding region of gene sets (orange) and in the whole genomic region (violet). ( b ) Phylogenetic relationships inferred based on the concatenated data set from universal single-copy genes. The number in the branches indicates the genome sizes. ( c ) Size expansion of genomic components of a homologous and syntenic locus between the locust and fly genome inferred from the Osiris genes, a conserved gene family across insects. ( d ) Deletion rates across five insect genomes that contain a substantial fraction of LTR retrotransposon copies. Because of their relaxed selection pressures and reputed neutral decay rates, LTR retrotransposon copies were used to estimate deletion rates. RepeatMasker searches were performed to determine the deletion rates of genomic retrotransposon copies using intact LTR retrotransposons as a query. The genomic visualization was created using the programme Circos. AGA, A. gambiae ; AME, A. mellifera ; API, A. pisum ; BMO, B. mori ; DME, D. melanogaster ; DPU, D. pulex ; LMI, L. migratoria ; NVI, Nasonia vitripennis ; PHU, P. humanus ; TCA, Tribolium castaneum ; . Full size image The total heterozygosity rate of the L. migratoria genome, which is the portion of heterozygous single-nucleotide polymorphisms between the two haploid components in the diploid genome, was estimated to be 1.15 × 10 −3 . We also observed a heterogeneous distribution of heterozygosity rates ( Fig. 1a , track b), which possibly resulted from inbreeding [18] . The possible reasons are the existence of alleles, which are homozygous lethal and the variation of recombination rates between different genomic regions [19] , [20] . We assessed the integrity and quality of the genome assembly using multiple evaluation methods ( Supplementary Figs S4 and S5 , and Supplementary Tables S4–S7 ). On the basis of these analyses, our assembly provides a good representation of the L. migratoria genome and is of suitable quality for subsequent analysis. Genome annotation and evolutionary analysis We annotated the genome and predicted 17,307 gene models by combining de novo prediction and evidence-based searches using four sequenced insect reference gene sets ( Drosophila melanogaster , Apis mellifera , Acyrthosiphon pisum and Pediculus humanus ), L. migratoria expressed sequence tags (ESTs) and RNA-seq data from transcriptomes that we created previously and for this work from multiple organs and developmental stages ( Supplementary Methods and Supplementary Table S8 ). We found that 93.8% of gene models showed expression (reads per kb per million mapped reads >1 in at least one sample). Of the inferred proteins, 74.9% matched entries in the NR, SWISS-PROT, InterPro or TrEMBL databases ( Supplementary Table S9 ). We identified over 2,639 repeat families using RepeatModeler; however, the top ten repeat families only represented ~10% of the total genome sequences, indicating there were no dominant families in the L. migratoria genome ( Supplementary Tables S10 and S11 ). The LINE RTE/BovB family, which has been documented in many species as having been acquired through an ancient lateral gene transfer event [21] , is the most prevalent repeat family (244 Mb, 4.05%) in the L. migratoria genome, and it may be still active as indicated by the presence of many full-length copies and intact protein domains [22] . The proliferation of a diverse range of repetitive elements is the main reason for the large size of the L. migratoria genome. Repetitive elements constituted ~60% of the assembled genome, of which DNA transposons (~24%) and LINE retrotransposons (17%) were the most abundant elements ( Fig. 1a , track c, Supplementary Note 1 and Supplementary Table S10 ). Among all transposons, DNA transposon exhibits the lowest divergent copies ( Fig. 1a , track d), which reflects their most recent invasions in the locust genome. On the basis of homologous regions of a conserved and syntenic Osiris gene family among insect orders [23] , we compared genomic components of L. migratoria with that of D. melanogaster ( Supplementary Fig. S6 ). The length of coding region has no difference, but the length of intronic, intergenic regions and repetitive elements in the L. migratoria genome is much larger than that of D. melanogaster ( Fig. 1c ). We compared the L. migratoria DNA deletion rates with that of five other insect genomes ( D. melanogaster , Anopheles gambiae , Bombyx mori , A. pisum and Aedes aegypti ) focusing on long terminal repeat retrotransposons, because these have neutral decay rates and easily identified complete structures [24] . We observed a positive correlation between DNA deletion and divergence of long terminal repeat copies ( P <0.01, Pearson’s correlation tests). The L. migratoria genome exhibits the lowest rate of DNA deletions relative to the other insects ( P <0.01, Wilcoxon tests; Fig. 1d ). These results are consistent with the previous reports and support the hypothesis that slow DNA loss contributes to genomic gigantism in animals [25] . The average intron length in the L. migratoria genome was 11,159 bp, which is >10 times longer than the average intron size of other insects and twice that of the average size in Homo sapiens ( Supplementary Table S8 and Supplementary Fig. S7 ). Pairwise comparison of intron sizes in nine insect species using one-to-one orthologous genes provided further support for this average size difference ( Supplementary Fig. S8 and Supplementary Table S12 ). We also carried out a genome-wide comparison of intron and genome size of 73 sequenced animal species and found that there was a positive correlation between average intron size and genome size ( P <0.01, Pearson’s correlation tests; Supplementary Fig. S9 ). The increased intron size in the L. migratoria genome compared with the other insects may partly be attributed to transposable element invasion ( Supplementary Fig. S10 ). Relative to this, we compared several other intron characteristics of the L. migratoria genome with other animal species ( Supplementary Note 1 ) and found that the U12-type intron (minor-class intron) number and the ratio of ratcheting point sites of L. migratoria are similar to those in vertebrates rather than insects ( Supplementary Figs S11 and S12 ). Previous reports have indicated that most insects have an enrichment of ratcheting point sites to allow for efficient splicing of long introns, whereas vertebrates use repetitive elements to aid in splicing long introns [26] . Our data here indicate that there may be convergent evolution of the splicing mechanisms associated with genome size expansion in animals. We used a maximum likelihood method for genome-scale phylogenetic analysis using 122 single-copy genes from 10 sequenced arthropod genomes ( Fig. 1b and Supplementary Fig. S13 ). The phylogenetic analysis revealed that the locust is the basal taxon for the other insects sequenced so far, and supports the paraphyletic status of the hemimetabolous insect species. Given the distinct developmental differences between hemimetabolous and holometabolous insects, we identified metamorphosis-specific gene sets, of which a large number of genes were related to the regulation of developmental processes ( Supplementary Table S13 ). A gene gain/loss analysis of these insect genomes showed a gain of about 55 new gene families in the lineage leading to L. migratoria ( Supplementary Fig. S13 ). Twenty-five significantly expanded gene families in the L. migratoria genome were mainly involved in detoxification, chemoreception, chromosome activity and nutritional metabolism, indicating unique adaptation features of the L. migratoria genome ( Supplementary Table S14 ). Phase change analysis Phase change is the defining characteristic of locust biology because of its critical roles in swarm formation ( Fig. 2a ) [5] . As a fascinating type of phenotypic plasticity, phase change is required to achieve biological complexity at all levels of biological organization, from molecules to large aggregation. Recent studies have highlighted the importance of DNA methylation for understanding insect phenotypic plasticity and biological complexity [27] , [28] , [29] . To investigate the potential involvement of epigenetic regulation in locust phase change, we performed a comparative methylome analysis for brain tissues between solitarious and gregarious locusts by a reduced representation bisulphite sequencing (RRBS) technology and then conducted a comparative transcriptome analysis for brain tissues over two time courses (within 64 h): starting at the onset of crowding of solitarious locusts and the isolation of gregarious locusts. 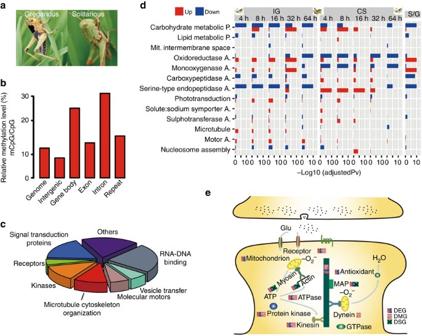Figure 2: Transcriptome and methylome analysis of locust phase change. (a) Locust phase polyphenism. The solitarious phase individual is relatively inactive and cryptically coloured, but gregarious phase individual actively swarms and is conspicuously coloured. (b) Relative CG methylation level of different genomic regions through a RRBS method. The ratio was defined as the number of methylated CG to the number of total CG, and was calculated using the CG on the reads that map to the defined regions. The results were derived from the data of brain samples of fourth-instar locust nymphs. (c) Functional classification of differentially methylated genes (DMGs) of brain tissues between solitarious and gregarious fourth-instar female nymphs. Genes with at least four differentially methylated CG sites were thought of as DMGs. (d) Gene ontology enrichment of differentially expressed genes (DEGs) in brain tissues of fourth-instar locust nymphs over time for the gregarization (crowding of solitarious locusts (CS)) and solitarization (isolation of gregarious locusts (IG)) processes (4, 8, 16, 32 and 64 h) compared with controls. The rightmost column denotes the comparison between the solitarious and gregarious control. The up- and downregulated genes are coloured as red and blue, respectively. The length of the bar denotes the −log10 of the adjustedP-value of the enrichment significance (Fisher’s exact test orχ2-test). A, activity; Mit, mitochondrion; P, process. (e) Model for molecular regulation of synaptic plasticity involved in locust phase change. In this model, DEGs, DMGs or differentially spliced genes (DSGs) were found for different components. MAP, microtubule-associated protein. Figure 2: Transcriptome and methylome analysis of locust phase change. ( a ) Locust phase polyphenism. The solitarious phase individual is relatively inactive and cryptically coloured, but gregarious phase individual actively swarms and is conspicuously coloured. ( b ) Relative CG methylation level of different genomic regions through a RRBS method. The ratio was defined as the number of methylated CG to the number of total CG, and was calculated using the CG on the reads that map to the defined regions. The results were derived from the data of brain samples of fourth-instar locust nymphs. ( c ) Functional classification of differentially methylated genes (DMGs) of brain tissues between solitarious and gregarious fourth-instar female nymphs. Genes with at least four differentially methylated CG sites were thought of as DMGs. ( d ) Gene ontology enrichment of differentially expressed genes (DEGs) in brain tissues of fourth-instar locust nymphs over time for the gregarization (crowding of solitarious locusts (CS)) and solitarization (isolation of gregarious locusts (IG)) processes (4, 8, 16, 32 and 64 h) compared with controls. The rightmost column denotes the comparison between the solitarious and gregarious control. The up- and downregulated genes are coloured as red and blue, respectively. The length of the bar denotes the −log10 of the adjusted P -value of the enrichment significance (Fisher’s exact test or χ 2 -test). A, activity; Mit, mitochondrion; P, process. ( e ) Model for molecular regulation of synaptic plasticity involved in locust phase change. In this model, DEGs, DMGs or differentially spliced genes (DSGs) were found for different components. MAP, microtubule-associated protein. Full size image We first assessed the DNA methylation patterns of the L. migratoria genome. We examined the distribution of observed/expected CpG content (CpG O/E ), which is a good measure of inferring the pattern of DNA methylation [30] , in the whole genome and observed that the CpG O/E of the coding region is lower and more fluctuated compared with those observed from the whole genomic region ( Fig. 1a , track e). A bimodal peak is clearly found in the CpG O/E obtained from the L. migratoria coding regions ( Supplementary Fig. S14 ). Furthermore, the L. migratoria genome seems to have a functional CpG methylation system, including two copies of Dnmt1 and one copy of Dnmt2 and Dnmt3 ( Supplementary Table S15 ). This is consistent with the patterns observed in researches on methylation in A. mellifera and A. pisum [31] , suggesting that L. migratoria likewise has a large proportion of genes that may be methylated. Through a low-pass bisulphite sequencing and RRBS ( Supplementary Fig. S15 ), we roughly estimated that 1.6% of genomic cytosines are methylcytosines. Nearly all the methylcytosines were located in CpG dinucleotides, which were substantially enriched in gene bodies ( Supplementary Figs S16 and S17 , and Supplementary Tables S16 and S17 ). Interestingly, we find that repetitive elements are highly methylated and introns have higher methylation levels than exons ( Fig. 2b ), which is different in other insect species where exons have higher methylation levels [32] . Hence, the L. migratoria genome probably represents a unique DNA methylation pattern existing in ancestral branches of insecta. Through RRBS, we found a total of 9,311,972 CpG sites that cover 11,743 genes ( Supplementary Table S18 ). Over 90 genes showed significant methylation differences between solitarious and gregarious locusts, and these were mainly classified into seven categories, including microtubule cytoskeleton organization, molecular motors, kinases, receptors, vesicle transfer, signal transduction proteins and RNA–DNA binding (Fig. 2c , Supplementary Fig. S18 and Supplementary Table S19 ). Many of these categories had been documented in various animal species to have a crucial role in neuronal functions connected to synaptic plasticity [33] , [34] . To further elucidate neuronal mechanisms underlying locust phase change, we conducted a series of transcriptome analyses of brain tissues from locust nymphs experiencing short-term solitarization and gregarization. We identified a total of 4,893 differentially expressed genes in at least one of the time points during both processes, and this accounted for 28.3% of the gene sets ( Supplementary Table S20 and Supplementary Fig. S19 ). Gene ontology (GO) analyses showed these fell into a variety of categories ( Supplementary Fig. S20 ), indicating that phase change induced a broad range of changes in CNS gene expression. GO enrichment analysis revealed that there were waves of gene expression changes occurring over the time courses of crowding of solitarious locusts and isolation of gregarious locusts ( Supplementary Tables S21 and S22 ) and that there were distinct temporal patterns for a number of genes ( Fig. 2d ). As a whole, during locust crowding, the genes associated with synaptic transmission, carbohydrate metabolism and nucleosome assembly displayed higher expression levels, whereas the expression levels of genes associated with oxidoreductase and antioxidase, microtubule and motor activity showed decreased expression. The expression patterns of these genes were reversed during gregarious locust isolation. These results suggest that crowding of solitarious locusts may trigger an increase in neuronal activity with a simultaneous suppression of antioxidative responses in the CNS during the onset of phase change in locusts. Alternative pre-messenger RNA splicing (AS) has an important role in development and phenotypic plasticity [35] . On the basis of the RNA-seq data from different developmental stages and tissues of the L. migratoria , we identified 168,646 splice junctions and showed that alternative 3′-splicing is the most prevalent form of AS ( Supplementary Fig. S21 ). Comparative AS transcript analysis revealed 45 genes that have differentially expressed isoforms between solitarious and gregarious locusts ( Supplementary Table S23 ). These include several genes implicated in cytoskeleton dynamics, for example, microtubule-associated protein futsch , ankyrin repeat domain-containing protein, neurofilament, myosin, calcium-transporting ATPase and Arrestin. It is noteworthy that the genes involved in the regulation of the cytoskeletal microtubular system were highlighted from the analysis of methylome, transcriptome and AS, respectively ( Fig. 2e ). Microtubules are essential structures for stable neuronal morphology and have important roles in neuronal polarization, development and plasticity [36] , [37] . Neuronal plasticity has been demonstrated to occur between solitarious and gregarious locusts accompanying behavioural change. Our results suggested that phase change is associated with multiple molecular processes involved in the regulation of microtubule dynamics in the locust CNS. Long-distance flight trait analysis The capacity of long-distance flight is the most distinguishing feature of L. migratoria [38] . Insect flight capacity depends on several factors, including wing and muscle morphology, neuroendocrine regulation and energy metabolism [39] . We annotated genes that are potentially relevant to these morphological features and physiological processes ( Supplementary Note 2 , Supplementary Tables S24–S31 and Supplementary Fig. S22 ) and compared the RNA-seq data derived from fat body tissues of locust adults after 2 h of flight and no flight ( Fig. 3 ). 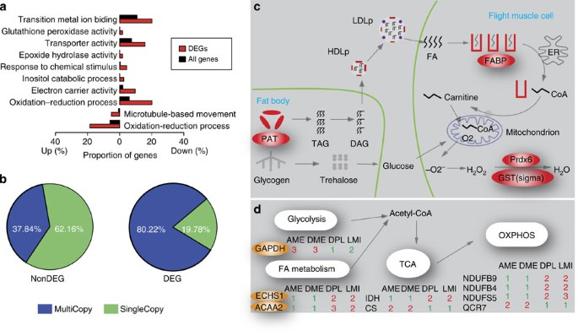Figure 3: Expansion of genes putatively involved in energy consumption duringL. migratoriaflight. (a) Overrepresented GO annotations for 472 differentially expressed genes (DEGs) in the fat body after 2 h of flight. The bar represents the proportion of the genes of one GO term in the DEGs (red) and all annotated genes (black). (b) Proportion of multi-copy (blue) and single-copy (green) genes for DEGs (right) and non-DEGs (left), respectively. (c) Expanded genes (red) involved in energy mobilization processes in theL. migratoriagenome. PAT, perilipin; TAG, triacylglycerol; DAG, diacylglycerol; FA, fatty acid; ER, endoplasmic reticulum; FABP, fatty-acid-binding protein; Prdx6, 9 I cysteine peroxiredoxins; GST, glutathione S-transferase. (d) Gene copy number variation in energy-related metabolic pathways between two insect species,A. mellifera(AME) andD. melanogaster(DME), which primarily use glucose as an energy source during flight, and two insect species,D. plexippus(DPL) andL. migratoria(LMI), which primarily use fatty acids. ACAA2, acetyl-CoA acyltransferase 2; TCA, tricarboxylic acid cycle; CS, citrate synthase; ECHS1, enoyl-CoA hydratase; GAPDH, glyceraldehyde 3-phosphate dehydrogenase; IDH, isocitrate dehydrogenase; NDUFB9, NADH dehydrogenase (ubiquinone) 1β subcomplex 9; NDUFB4, NADH dehydrogenase (ubiquinone) 1β subcomplex 4; OXPHOS, Oxidative phosphorylation; NDUFS5, NADH dehydrogenase (ubiquinone) Fe-S protein 5; and QCR7, ubiquinol–cytochromecreductase subunit 7. Figure 3: Expansion of genes putatively involved in energy consumption during L. migratoria flight. ( a ) Overrepresented GO annotations for 472 differentially expressed genes (DEGs) in the fat body after 2 h of flight. The bar represents the proportion of the genes of one GO term in the DEGs (red) and all annotated genes (black). ( b ) Proportion of multi-copy (blue) and single-copy (green) genes for DEGs (right) and non-DEGs (left), respectively. ( c ) Expanded genes (red) involved in energy mobilization processes in the L. migratoria genome. PAT, perilipin; TAG, triacylglycerol; DAG, diacylglycerol; FA, fatty acid; ER, endoplasmic reticulum; FABP, fatty-acid-binding protein; Prdx6, 9 I cysteine peroxiredoxins; GST, glutathione S-transferase. ( d ) Gene copy number variation in energy-related metabolic pathways between two insect species, A. mellifera (AME) and D. melanogaster (DME), which primarily use glucose as an energy source during flight, and two insect species, D. plexippus (DPL) and L. migratoria (LMI), which primarily use fatty acids. ACAA2, acetyl-CoA acyltransferase 2; TCA, tricarboxylic acid cycle; CS, citrate synthase; ECHS1, enoyl-CoA hydratase; GAPDH, glyceraldehyde 3-phosphate dehydrogenase; IDH, isocitrate dehydrogenase; NDUFB9, NADH dehydrogenase (ubiquinone) 1β subcomplex 9; NDUFB4, NADH dehydrogenase (ubiquinone) 1β subcomplex 4; OXPHOS, Oxidative phosphorylation; NDUFS5, NADH dehydrogenase (ubiquinone) Fe-S protein 5; and QCR7, ubiquinol–cytochrome c reductase subunit 7. Full size image Most of 472 differentially expressed genes related to flight were enriched into several GO categories involved in energy metabolism ( Fig. 3a ) and have more duplicated copies compared with non-differentially expressed genes ( χ 2 -test, P <1e−16; Fig. 3b ). Through a comparison with nine other sequenced insects, we observed significant copy number expansion in genes associated with lipid mobilization and antioxidant protection in the L. migratoria genome, including 7 perilipins, 11 fatty-acid-binding proteins, 9 I cysteine peroxiredoxins (Prdx6s) and 12 sigma glutathione S -transferase (GST) genes ( Fig. 3c , Supplementary Figs S23–S24 , and Supplementary Tables S28 and S30–32 ). Perilipins are predominantly located on the surface layer of intracellular lipid droplets in adipocytes [40] and have a critical role in lipid accumulation [41] . fatty-acid-binding proteins are known to be directly correlated with the metabolic rate in locust flight muscle tissues, and thus may contribute to the extremely high metabolic rate of fatty acid oxidation for energy generation [42] . The two antioxidant gene families, Prdx6 and sigma GST, are involved in protection against reactive oxygen species damage caused by flight activity [43] . Furthermore, several members of these families were differentially expressed in the fat body tissues before and after flying, indicating their important roles in the flying process ( Supplementary Fig. S25 ). Given that flight is considered one of the most energy-demanding exercises in insects [44] , the expansion of genes involved in lipid metabolism indicate that L. migratoria has developed a highly efficient energy supply system to fulfill the intensive energy consumption during their long-distance flight [45] . Different insects use different fuel sources to provide energy during flight [46] . For example, A. mellifera and D. melanogaster primarily use carbohydrates, whereas Danaus plexippus and L. migratoria mainly use lipids during long-distance flight [47] . To investigate whether the energy metabolic pathways undergo changes owing to the need for different fuel source preferences, we compared the copy number variation of genes involved in carbohydrate and lipid metabolism. We found that there were more copies of glycolytic gene glyceraldehyde 3-phosphate dehydrogenase in A. mellifera and D. melanogaster , whereas there were more copies of enoyl-CoA hydratase and acetyl-CoA acyltransferase 2 in D. plexippus and L. migratoria ( Fig. 3d ). It is interesting to note that enoyl-CoA hydratase and acetyl-CoA acyltransferase 2 belong to a multi-enzyme complex located in the inner mitochondrial membrane that catalyse two distinct steps of β-oxidation cycle of fatty acid degradation [48] . Therefore, these two enzymes need be functionally tightly associated to allow efficient substrate channelling from one active site to the next. The increase of gene copies involved in L. migratoria and D. plexippus in fatty acid degradation process is likely to serve as an adaptation for the preference of lipids as energy source during long-distance flight. Feeding trait analysis L. migratoria usually prefer gramineous plants (grasses) as a food source, which includes the majority of crop species [49] . Food selection processes are primarily mediated by the detection of chemical cues and the ability of an insect to handle plant toxins [50] . We identified four multigene families putatively related to the detection of plant odours in the L. migratoria genome by carrying out similarity searches using information from known insect protein sequences ( Supplementary Note 2 ). These families included 22 odourant-binding proteins, 95 olfactory receptors, 75 gustatory receptors and 10 ionotropic receptors ( Fig. 4a ). We found that gustatory receptor and olfactory receptor gene families have undergone locust-specific expansion ( Supplementary Figs S26 and S27 ), which might reflect their strong adaptation for ecological specialization related to host plant recognition. 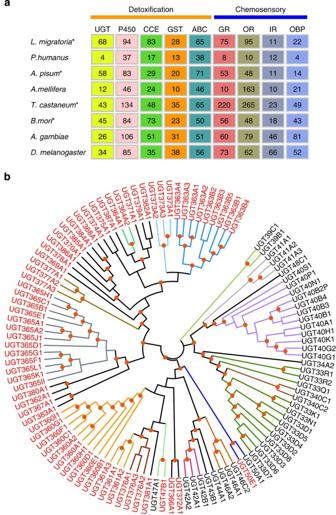Figure 4: Gene families putatively related toL. migratoriahost plant adaptation. (a) Numbers of detoxification-related and chemosensory-related genes in the genomes of eight selected insects. *Herbivorous insects. UGT, UDP glycosyltransferases; CCE, carboxyl/choline esterases; GST, glutathione S-transferase; ABC, ATP-binding cassette; GR, gustatory receptor; OR, odorant receptor; IR, ionotropic receptor; OBP, odorant-binding protein. (b) The phylogenetic relationship of the different UGT families. Family members in red are fromL. migratoriaand those in black are from other insects. Nodes with >70% bootstrap support (100 replicates) are indicated in orange circles. UGTs are named after the standard UGT nomenclature guide. For clarity, we show only a selected number of representatives from the UGT families because of the large number of UGT families identified. Figure 4: Gene families putatively related to L. migratoria host plant adaptation. ( a ) Numbers of detoxification-related and chemosensory-related genes in the genomes of eight selected insects. *Herbivorous insects. UGT, UDP glycosyltransferases; CCE, carboxyl/choline esterases; GST, glutathione S-transferase; ABC, ATP-binding cassette; GR, gustatory receptor; OR, odorant receptor; IR, ionotropic receptor; OBP, odorant-binding protein. ( b ) The phylogenetic relationship of the different UGT families. Family members in red are from L. migratoria and those in black are from other insects. Nodes with >70% bootstrap support (100 replicates) are indicated in orange circles. UGTs are named after the standard UGT nomenclature guide. For clarity, we show only a selected number of representatives from the UGT families because of the large number of UGT families identified. Full size image We also found that five of the known gene families putatively involved in detoxification enzymes and xenobiotic transporters in the locust had a unique composition and were expanded in L. migratoria . We identified 68 UDP glycosyltransferases (UGTs), 80 carboxyl/choline esterases, 94 cytochrome P450s, 28 GSTs and 65 ATP-binding cassette transporters ( Supplementary Tables S32–S34 and Supplementary Figs S28–S32 ). Substantial expansion occurred in the UGT and carboxyl/choline esterase families, representing the largest family expansion in any insect genome sequenced so far ( Fig. 4b ). The expansion of multi-detoxification gene families suggests that L. migratoria has an all-purpose detoxification system, allowing it to handle a broad range of secondary metabolites present in their host plants [51] . Interestingly, we also found that the repertoires of the UGT gene family from four herbivorous insects far exceeded the numbers found in the non-herbivorous insects ( Fig. 4a ). Insect UGTs are involved in glucosidation, which has a major role in the inactivation and excretion of a variety of toxic plant secondary metabolites, including alkaloids, phenols and flavonoids, which are present in substantial amounts in gramineous plants [52] , [53] . Identification of gene targets for pest control Locust plague control urgently requires safe and effective new insecticides or other solutions [2] . We therefore searched the L. migratoria genome for insecticide gene targets. We identified 34 cys-loop ligand-gated ion channels and 90 G-protein-coupled receptors, which are considered to be major traditional insecticide targets [54] , [55] ( Supplementary Note 3 and Supplementary Table S35 ). Using in-silico screening [56] for L. migratoria orthologues of Caenorhabditis elegans and D. melanogaster lethal genes (linked to lethal phenotypes on gene perturbation), we identified 166 genes that may be worth considering for targets in alternative pest control strategies given that they are single copy, have lower allelic variability and lack similarity to human genes. Among these genes, several have been reported as successful targets in previous studies, and include kinases, ATPases, synthases, carboxylesterases and receptors [57] . We also identified the gene repertoire of several biological processes that may serve as mechanistic targets and lead to the development of specific and sustainable pest control methods [58] , including the immune system, RNA interference pathway and cuticle metabolism ( Supplementary Tables S36–S40 ). Our analysis indicates that a massive number of repetitive elements (at least 60%) exist in the L. migratoria genome and their rates of loss are lower than those in other insect species. This partially explains the large genome size in L. migratoria . Comparative genomic analysis revealed locust-specific expansions of many gene families, particularly those that are involved in energy consumption and detoxification, suggesting a genomic basis for long-distance flight capacity and phytophagy of locusts. The analyses of the methylome and transcriptome revealed the complex molecular regulation of phase change involving extensive participation of DNA methylation, transcription and alternative splicing in the CNS. The information from the L. migratoria genome, transcriptome and methylome obtained in this study serves as a major step towards better understanding of the locust plague outbreaks. It not only enables us to combat against this distractive event but also increase the use of this species as a model system in biological and biomedical research. Sample collection and genome sequencing The strain for genome sequencing originated from inbred laboratory strains of solitarious locusts, which were produced from eight generations of sib mating at the Institute of Zoology, CAS, China. DNA for genome sequencing was extracted from the whole body of one female adult, with the exception of its guts. Genomic DNA was isolated using standard molecular biology techniques. Gradient increased insert-size libraries, 170, 200, 500 and 800 bp and 2, 5, 10, 20 and 40 kb were constructed. All libraries were sequenced on Illumina HiSeq 2000. In total, 42 paired-end sequencing libraries were constructed and 82 lanes were sequenced, producing 1,135 Gb of raw data. Further low-quality and duplicated reads filtering resulted in 720 Gb (114 × coverage) data for genome assembly ( Supplementary Table S1 ). Genome assembly For quality control, raw data was filtered for PCR duplication, adaptor contamination and low quality. After filtering, 721 Gb (or 114.4 × ) of data were retained for assembly. SOAPdenovo [17] was selected to assemble the L. migratoria genome. The paired-end reads of short insert-size libraries were used to construct contigs, and those of long insert-size libraries were used to connect contigs and generate scaffolds. All the reads were used to fill gaps in the scaffolds. On the basis of our tests of multiple combinations of assembly parameters, ‘–K 43 –M 3’ was chosen in the final assembly. Approximately 350.95 Gb (or 50.1 × ) of data was used to build contigs, and all high-quality data were used to build scaffolds. Contigs and scaffolds <200 bp long were filtered out. The final total contig size and N50 were 5.95 Gb and 9.26 kb, respectively. The total scaffold size and N50 were 6.74 Gb and 281.75 kb, respectively. The total length of assembled sequences is ~400 Mb larger than the genome size estimated by the flow cytometry and 17-mer analysis. To determine whether heterozygosity contributes to redundancy in assembled sequences, ~22 × paired-end reads with 200 bp inserts were mapped to the assembled sequences using MAQ-0.7.17 (ref. 59 ) with default parameters, except –C 1. Whole-genome coverage depth distribution revealed a peak at half of the expected average coverage depth, ~11 × (half depth), which may have resulted from the heterozygosity. To reduce redundancy, we first identified all regions with half depth using the following criteria: length>200 bp, average depth<15 × and >95% of the positions have <15 × depth. Next, all the scaffolds with half depth were aligned self-to-self using BLAT with identity >90%. The overlapped terminal region of the shorter scaffold was removed if the overlapping regions had half depth and at least one of the four terminal lengths was <2 kb long. Contamination of bacterial and viral DNA sequences was also removed. All assembled sequences were aligned to the genome sequences of viruses and bacteria available through NCBI. Aligned sequences with >90% identity and longer than 200 bp were filtered out from the final assembly. To minimize any negative influence of filtering, assembled sequences covered by an EST sequence were retained. Our de novo assembly approaches combined with the filtering steps resulted in a final genome assembly of 6.52 Gb with contig N50 9.3 kb ( Supplementary Table S3 ). The assembly was further improved to a final scaffold N50 323 kb using the gene-scaffold method by combining evidence from RNA-seq data and homologous genes ( Supplementary Methods ). Linkage mapping of scaffolds We used 106 F1 individuals produced from a cross between two L. migratoria , one from the Hainan province and another from the laboratory-raised population, to perform RADseq. BWA (v. 0.6.2) was used to align the reads to the reference. SAMtools (v. 0.1.18) [60] were used to call single-nucleotide polymorphism and filtering. A custom PERL script was developed to identify segregating polymorphic patterns and classify linkage groups. Marker ordering and spacing were carried out using JoinMap (v. 3.0) [61] . Protein coding gene annotation For homology-based prediction, Genewise was used to improve gene models that acquired from the protein sets of four insects. For de novo prediction, Augustus [62] , SNAP [63] and Glimmer-HMM [64] were employed on the repeat masked-assembly sequences. RefSeq proteins from A. pisum and P. humanus were used as training data to obtain suitable parameters in the L. migratoria gene prediction. For transcriptome-based prediction, PASA [65] was used to define gene structures from 45,436 ESTs, and TopHat and Cufflinks were used to obtain transcript structures from RNA-seq data that were collected from various developmental stages. Finally, GLEAN [66] was used to merge the evidences from homology-based, de novo -derived and transcript gene sets to form a comprehensive and non-redundant reference gene set. After filtering and manual curation, 17,307 genes were obtained ( Supplementary Table S8 and Supplementary Methods ). Gene family analysis Orthology analysis was carried out by the TreeFam [67] pipeline using nine insects and Daphnia pulex . The rate and direction of gene family size in L. migratoria and its related species were inferred using CAFÉ [68] ( Supplementary Methods ). Transcriptome sequencing Samples for RNA-seq were prepared from a mixed samples of various developmental stages and ten tissues of gregarious adults and brain tissues of fourth-instar nymphs undergoing time courses of gregarization and solitarization ( Supplementary Methods ). Total RNA was extracted using the TRIzol reagent (Invitrogen) and treated with RNase-free DNase I. Poly(A) mRNA was isolated using oligo dT beads. First-strand complementary DNA was generated using random hexamer-primed reverse transcription, followed by synthesis of the second-strand cDNA using RNaseH and DNA polymerase I. Paired-end RNA-seq libraries were prepared following Illumina’s protocols and sequenced on the Illumina HiSeq 2000 platform. To assist gene annotation, a cDNA library with mixed samples from various organs and developmental stages was constructed, and was then normalized by the duplex-specific nuclease method followed by cluster generation on the Illumina HiSeq 2000 platform. This method could reduce expression redundancy and facilitate novel gene discovery. Gene expression analysis The RNA-seq reads were mapped using Tophat. Gene expression levels were measured using the reads per kb per million mapped reads criteria. To minimize the influence of differences in RNA output size between samples, the numbers of total reads were normalized by multiplying with normalization factors as suggested by Robinson and Oshlack [69] . Differentially expressed genes were detected using the method described by Chen et al . [70] , which was constructed based on Poisson distribution and eliminated the influences of RNA output size, sequencing depth and gene length. Reduced representation bisulphite sequencing Solitarious and gregarious locusts were reared as described in a previous publication [11] . Brain tissues of 3-day-old fourth-instar gregarious and solitarious females were dissected and placed in liquid nitrogen. Each sample contained 100 brain tissues. DNA was extracted using the Gentra puregene Kit (Qiagen, USA). Next, 5 μg of genomic DNA was digested with 300 U of the Msp I enzyme (New England Biolabs, USA) in 100 μl reactions at 37 °C for 16–19 h. After purification, the digested products were subjected to blunt ending, dA addition and methylated-adapter ligation. To obtain DNA fractions of 40–120 bp and 120–220 bp ranges of Msp I-digested products, two ranges of 160–240 bp and 240–340 bp adapter-ligated fractions were excised and purified from a 2% agarose gel. Bisulphite conversion was conducted using the ZYMO EZ DNA Methylation-Gold Kit (ZYMO) following the manufacturer’s instructions. The same bisulphite conversion was also conducted for one sample that was not digested by Msp I. The final libraries were generated by PCR amplification of 11–13 cycles using JumpStart Taq DNA Polymerase (Sigma). After testing using an Agilent 2100 Bioanalyzer (Agilent Technologies) and real-time PCR, the libraries were analysed on the HiSeq 2000 system. In total, 13.5 Gb and 12.8 Gb of data were produced for gregarious and solitarious samples, respectively. To validate the methylation level, 63 TA clones (26 in 120–220 bp and 37 in 40–120 bp) were sequenced by bisulphite PCR using the Sanger method. A methylation ratio of 3.42% was detected for the CG sites. Accession codes : Assembled genome sequences for Locusta migratoria have been deposited in DDBJ/EMBL/GenBank nucleotide core database under accession code AVCP000000000 . Genome sequence reads and RRBS methylation sequence reads have been deposited in the GenBank sequence read archive under accession codes SRA064067 and SRA067627 , respectively. How to cite this article: Wang, X. et al . The locust genome provides insight into swarm formation and long-distance flight. Nat. Commun. 5:2957 doi: 10.1038/ncomms3957 (2014).